Defect-induced plating of lithium metal within porous graphene networks Lithium metal is known to possess a very high theoretical capacity of 3,842 mAh g −1 in lithium batteries. However, the use of metallic lithium leads to extensive dendritic growth that poses serious safety hazards. Hence, lithium metal has long been replaced by layered lithium metal oxide and phospho-olivine cathodes that offer safer performance over extended cycling, although significantly compromising on the achievable capacities. Here we report the defect-induced plating of metallic lithium within the interior of a porous graphene network. The network acts as a caged entrapment for lithium metal that prevents dendritic growth, facilitating extended cycling of the electrode. The plating of lithium metal within the interior of the porous graphene structure results in very high specific capacities in excess of 850 mAh g −1 . Extended testing for over 1,000 charge/discharge cycles indicates excellent reversibility and coulombic efficiencies above 99%. The first practical lithium (Li) battery was developed as far back as 1976 by Exxon, using TiS 2 as the anode and bare lithium metal as the cathode [1] . However, soon after its inception the viability of such a cell composition was questioned owing primarily to the use of the lithium metal–liquid electrolyte combination. In a non-aqueous electrolyte, dendritic projections tend to develop at the lithium–electrolyte interface [2] , [3] , [4] . The dendritic growth occurs during the charge/discharge cycling process, expanding in diameter and at the same time, extending from the tip ( Supplementary Fig. 1 ). The tip-wise extension poses a serious challenge as extended cycling can often cause the dendrite tip to pierce through the separator, resulting in an electrical short between the anode and cathode. Moreover, the tip-wise dendritic formation process is accelerated as the current density is increased (typically ≥0.1 C, where a rate of n C is defined as charge or discharge in 1/ n hours), which is attributed to a higher localized charge density at the dendrite tip. This in turn significantly limits the rate capability of such batteries. In order to overcome the challenges posed by dendritic growth in pure lithium metal cathodes, the battery community resorted to layered-structured frameworks of lithium compounds such as transitional metal oxides [5] , [6] , spinels [7] , [8] and phospho-olivines [9] , [10] as cathode materials for rechargeable lithium batteries. In 1980, Goodenough and co-workers [11] first demonstrated the use of LiCoO 2 as cathodes with a theoretical capacity of ~273 mAh g −1 and a theoretical energy density of 1.11 kWh kg −1 . However, the practical capacity [12] of LiCoO 2 is only ~140 mAh g −1 (with energy densities of ~500 Wh kg −1 ) due to the restricted cycling voltage window of 4.2 V. Cycling above 4.2 V results in the dissolution of cobalt in the electrolyte, thereby leading to a rapid decay in capacity. In order to overcome these drawbacks, various approaches have been adopted such as incorporation of coatings and partial substitution of cobalt with nickel, which helps suppress lattice expansion and hence allows for extended cycling [13] , [14] . Such advancements have ensured the success of LiCoO 2 cathodes; these materials are the most widely used in today’s commercial lithium-ion batteries. Anodes for lithium batteries on the other hand include a wide variety of hosts capable of electrochemical reactions with lithium such as formation of alloys or intercalates. Conventionally, graphite is the preferred anode material exhibiting an intercalation reaction with lithium to yield LiC 6 (corresponding to a theoretical capacity of 372 mAh g −1 ). The first such commercial lithium-ion cell constructed with a graphitic anode and LiCoO 2 cathode was developed in 1991 by Sony Corporation [15] . Since then, there have been significant advancements in the anode chemistry. One of the major thrusts has been in identifying anodes capable of accommodating more lithium ions and hence, delivering higher energy densities. More recently, there has been a significant effort in identifying composite anodes, especially of carbon–silicon, that can combine the stability and electrical conductivity of carbon with the high specific capacity of silicon [16] , [17] , [18] . This has enabled a steady capacity in excess of 1,000 mAh g −1 to be achieved over extended cycling. Compared with some of the recent advances that anodes have made in terms of stability and achievable capacities, cathode materials are still somewhat lagging behind. The unavailability of high-capacity and low-cost cathode materials that display stable response over extended cycling remains one of the key challenges to achieving breakthrough improvements in the energy density and performance of lithium-ion rechargeable batteries. In this study we demonstrate thermally reduced, free-standing porous graphene networks (PGN) as high-capacity anode as well as cathode materials in lithium-ion batteries. We demonstrate a new mechanism in which defects in the graphene lattice act as seed points that initiate plating of lithium metal within the interior of the porous graphene structure. This entrapment of lithium metal results in very high specific capacities and energy densities. When compared with graphitic anodes (commonly LiC 6 : capacity ~372 mAh g −1 , energy density ~180 Wh kg −1 ), the PGN delivers capacities of ~900 mAh g −1 with an energy density of ~547 Wh kg −1 . Compared with conventional cathodes (commonly LiCoO 2 : capacity~140 mAh g −1 , energy density ~518 Wh kg −1 ), the PGN structure with entrapped lithium metal provides capacities of ~850 mAh g −1 , with an energy density of ~637 Wh kg −1 . Extended testing for over 1,000 charge/discharge cycles indicates excellent reversibility and coulombic efficiencies above 99%. Importantly, even after 1,000 cycles there is no indication of any significant dendritic structures, since the lithium metal is caged within the pores of the PGN structure. We also demonstrate a full-cell configuration where PGN electrodes are used as both the anode and cathode and Li is reversibly plated and contained within the porous PGN structure. Such all-carbon electrodes could potentially offer an environmentally friendly solution that does not utilize hazardous materials such as Co in battery manufacturing. PGN synthesis and coin cell testing Synthesis of a free-standing (binder-free) PGN was performed by administering a thermal shock to graphene oxide (GO) paper, as shown schematically in Fig. 1a . The thermal shock treatment involved introducing a free-standing GO paper (~10-μm thick) into a tube furnace preheated to ~700 °C and filled with an inert argon atmosphere for a period of ~45 s. This induced a deoxygenation reaction in GO and the rapid outgassing resulted in the formation of pores measuring between a few nanometres to a few hundred nanometres. The as-obtained free-standing graphene paper was then assembled as an anode against a lithium foil in a half-cell configuration and cycled ( Fig. 1b ) between 3 V and 0.03 V at a rate of 1 C (current density of ~0.37 A g −1 ). Results at higher charge/discharge rates (10–150C) are provided in Supplementary Figs 2,3 . The initial capacity was measured to be ~600 mAh g −1 , which is much larger than the theoretical capacity of graphite. Interestingly, the capacity was observed to increase upon subsequent cycling. In fact, we observed a sustained rise over 300 charge/discharge cycles that increases the capacity by more than 150% before finally achieving a steady discharge capacity of ~915 mAh g −1 with an average coulombic efficiency as high as 99% ( Fig. 1b ). 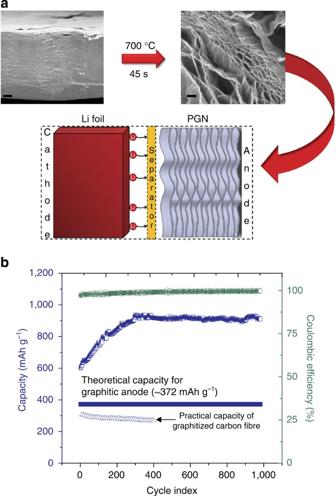Figure 1: PGN anodes for high-capacity lithium-ion batteries. (a) Reduction of GO paper by means of a thermal shock to produce a free-standing, PGN. The PGN is then assembled into a half-cell and tested as an anode material in lithium ion batteries. Scale bar in the left scanning electron microscopy image is 2 μm, while in the right image it is 200 nm. (b) Capacity and coulombic efficiency versus cycle index of the PGN anode. The PGN anode develops a maximum specific capacity of ~915 mAh g−1(~2.5 times higher than the theoretical capacity of graphite), with coulombic efficiencies above 99%. For comparison, the practical capacity of graphitic anodes has also been included19. The reason why such a porous graphene anode delivers a capacity and energy density ( Table 1 ) that is almost threefold higher than conventional graphitic anodes [19] and stable over 1,000 charge/discharge cycles remains unclear. Some studies with graphene anodes have reported achieving a capacity higher than the theoretical capacity of graphite and have generally attributed it to the formation of Li 2 C 6 , corresponding to the intercalation of lithium ions on both sides of the graphene sheets [20] , [21] . However, a detailed understanding of this phenomenon is fundamentally lacking at this point. Figure 1: PGN anodes for high-capacity lithium-ion batteries. ( a ) Reduction of GO paper by means of a thermal shock to produce a free-standing, PGN. The PGN is then assembled into a half-cell and tested as an anode material in lithium ion batteries. Scale bar in the left scanning electron microscopy image is 2 μm, while in the right image it is 200 nm. ( b ) Capacity and coulombic efficiency versus cycle index of the PGN anode. The PGN anode develops a maximum specific capacity of ~915 mAh g −1 (~2.5 times higher than the theoretical capacity of graphite), with coulombic efficiencies above 99%. For comparison, the practical capacity of graphitic anodes has also been included [19] . Full size image Table 1 Comparison of PGNs with conventional electrode materials. Full size table X-ray characterization studies To uncover the underlying mechanism(s) responsible for the results in Fig. 1b , we used X-ray photoelectron spectroscopy (XPS) to study the material composition of the PGN (the top surface of the PGN was partially removed by using the scotch tape method to expose the interior of the electrode for characterization purposes). Two anodes were characterized—one at the end of the 1,000 th lithiation step and another at the end of the 300 th delithiation step. The anodes were disassembled inside an argon-filled glove box with oxygen and moisture maintained at <0.1 p.p.m. The lithiated porous graphene anode showed a prominent lithium metal peak ( Fig. 2a ), thereby clearly indicating the presence of lithium metal within the porous graphene structure. By contrast, in the completely delithiated sample, the lithium metal peak was absent. This observation strongly suggests the participation of lithium metal in the charge/discharge reaction of the porous graphene anode. Interestingly, no peak was observed that could be attributed to LiC 6 , the standard intercalated state [22] in graphitic anodes. The absence of the LiC 6 signature in XPS suggests the existence of alternate mechanisms for lithium insertion within PGN anodes. The voltage profiles of the PGN anode (shown in Supplementary Figs 4–5 ) indicate that the capacity contribution from 3 V to 1.5 V during the lithiation step is merely ~11% of the total capacity. This suggests that redox reactions that take place in this voltage window between lithium and residual oxygen containing functional groups such as carbonyls are unlikely to be playing a significant role. 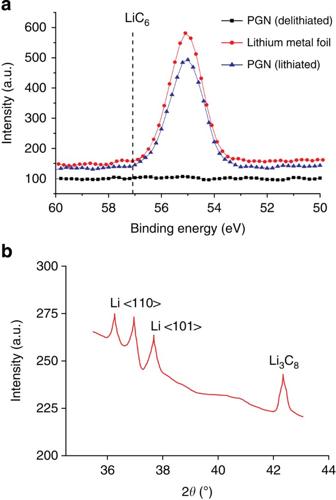Figure 2: X-ray characterization of the PGN structure. (a) X-ray photoelectron spectroscopy (XPS) Li 1 s scans of lithiated and delithiated PGN along with a bare lithium metal foil as the control. Lithiated PGN displayed a strong lithium metal peak that matches the signature from the metallic lithium foil, while no peaks were observed for LiC6, the conventional intercalation state in graphitic anodes. On the other hand, delithiated PGN displayed a contrasting absence of lithium metal, indicating excellent reversibility. The LiC6peak position is taken from ref.22. (b) X-ray diffraction (XRD) profile of lithiated PGN indicating prominent lithium metal peaks23along with a peak for Li3C8(ref.24). The unmarked peak is attributed to Li2CO3, a common component found in the solid electrolyte interphase (SEI), which is present presumably due to traces of un-removed SEI. Figure 2: X-ray characterization of the PGN structure. ( a ) X-ray photoelectron spectroscopy (XPS) Li 1 s scans of lithiated and delithiated PGN along with a bare lithium metal foil as the control. Lithiated PGN displayed a strong lithium metal peak that matches the signature from the metallic lithium foil, while no peaks were observed for LiC 6 , the conventional intercalation state in graphitic anodes. On the other hand, delithiated PGN displayed a contrasting absence of lithium metal, indicating excellent reversibility. The LiC 6 peak position is taken from ref. 22 . ( b ) X-ray diffraction (XRD) profile of lithiated PGN indicating prominent lithium metal peaks [23] along with a peak for Li 3 C 8 (ref. 24 ). The unmarked peak is attributed to Li 2 CO 3 , a common component found in the solid electrolyte interphase (SEI), which is present presumably due to traces of un-removed SEI. Full size image To further investigate the intercalation chemistry, X-ray diffraction (XRD) measurements were carried out on a completely lithiated graphene anode ( Fig. 2b ). Consistent with XPS, the XRD data also revealed strong lithium metal peaks corresponding to <110> and <101> crystal planes [23] , further confirming the participation of lithium metal in the charge/discharge reactions. Most interestingly, a strong peak for Li 3 C 8 was also observed [24] . This observation is striking as the presence of a lithium intercalated state with such a high lithium-to-carbon ratio has never been reported previously. The formation of Li 3 C 8 by itself can provide a maximum theoretical capacity of 837 mAh g −1 , which is competitive with other high-performance non-carbonaceous anodes such as silicon (4,200 mAh g −1 ), germanium (1,600 mAh g −1 ) and tin oxide (1,491 mAh g −1 ). It is to be noted here that lithiated graphitic anodes in general tend to show XRD peaks corresponding to stage I (LiC 6 ) and stage II (LiC 12 ) intercalations only. The absence of the LiC 6 signature ( Fig. 2b ) for PGN anodes can be attributed to the predominance of Li 3 C 8 and lithium metal plating as the primary and favourable reaction mechanisms. Ab initio modelling The first step in understanding the formation of Li 3 C 8 was to investigate the presence of defects in the graphene lattice and their participation in lithium ion interaction. Recent studies by transmission electron microscopy (TEM) [25] , [26] and scanning tunnelling microscopy (STM) [27] , [28] , [29] have discovered the existence of a variety of structural defects in graphene. While Stone–Wales defect (defect generated by pure reconstruction of a graphene lattice into non-hexagonal forms) is less likely to form in thermally reduced GO due to a high formation energy required for the incorporation of such a defect, the existence of vacancies is far more likely. Vacancies are primarily of two types—single vacancy and multiple vacancy. However, a single vacancy, arising from a missing lattice atom, is generally less stable owing to the presence of dangling bonds. A divacancy (DV) on the other hand is much more thermodynamically favourable over single vacancies and would thus be more likely to exist [30] , [31] . In fact, experiments indicate that DV defects are highly prevalent in GO sheets reduced by the thermal shock method, which is also consistent with simulation results [32] , [33] . To understand the role of defects, we performed first-principle density functional theory (DFT) calculations to study lithium interaction with graphene. Initially, lithium adsorption in pristine graphene was investigated ( Supplementary Fig. 6 ) before studying the nature of adsorption in graphene with DV defects. The lattice constant of graphene and the initial distance between the graphene plane and lithium are 2.4640 Å and 2.006 Å, respectively [34] . Two sites for lithium adsorption were considered: the site on the top of a carbon atom and the site in the centre of a hexagon. The potential for lithium adsorption on to the pristine graphene lattice was measured for different lithium concentrations and were found to be negative in value ( Supplementary Fig. S7 ), implying that lithium adsorption is not possible in pristine graphene and hence lithium atoms can only intercalate into (and occupy) the empty spaces between the graphene planes [35] . The packing density of Li atoms is dictated by the Li-to-Li and Li-to-graphene van der Waals interactions—this typically results in LiC 6 , the standard intercalated state of lithium in graphitic anodes (with a theoretical capacity of 372 mAh g −1 ). Next, a DV defect was incorporated by removing a C–C dimer from perfect graphene ( Fig. 3a ). Lithium adsorption was studied in three different locations: centre of defect, adjacent to the defect and far from the defect. The lithiation potential was subsequently observed to be the highest (0.7415, eV) at the centre of defect while dropping to about half (0.3658, eV) at the location farthest from the defect, indicating that the defective zone was the most favourable site for lithium adsorption. Finally, five different percentages of DV defects (6.25, 12.50, 16, 18.75 and 25%) were considered and the prospective nature of their intercalation with lithium atoms was compared with the experimentally obtained observation of Li 3 C 8 formation. All the systems shown here are the relaxed structures. For each percentage of defects, DFT calculations were carried out for different lithium concentration until the maximum limit for capacity was obtained, that is, when a negative lithiation potential was reached. When lithium is distributed on and around the defective sites, the tendency for adsorption was found to increase significantly. For instance, for a 12.5% DV defect density, the maximum capacity is ~400 mAh g −1 with potential of ~0.05 eV. As the defect density was increased, the maximum capacity was also found to increase—for example, a 16% DV defect density contributed towards a capacity of ~585 mAh g −1 with a potential range of 1–1.5 eV. 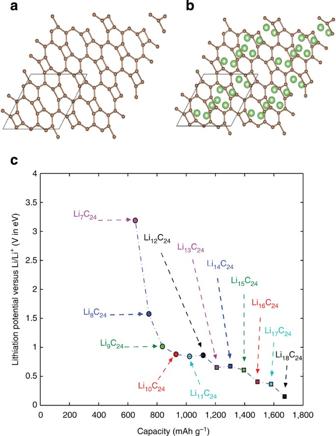Figure 3: Theoretical study of defect-induced intercalation of lithium in graphene. (a) Graphene lattice with 25% DV defects. (b) Lithium is found to adsorb strongly to such DV defects in stable configurations. This particular configuration is for Li3C8. (c) Capacity (mAh g−1) versus lithiation potential (eV) for 25% DV defects in graphene. Figure 3: Theoretical study of defect-induced intercalation of lithium in graphene. ( a ) Graphene lattice with 25% DV defects. ( b ) Lithium is found to adsorb strongly to such DV defects in stable configurations. This particular configuration is for Li 3 C 8 . ( c ) Capacity (mAh g −1 ) versus lithiation potential (eV) for 25% DV defects in graphene. Full size image However, a study on the highest defect density, that is, 25% indicates the possibility of achieving extraordinarily high capacities. It is to be noted here that 25% DV defect is the maximum limit for the presence of such a defect beyond which there will be dangling bonds of carbon atoms. For the highest-percentage DV defect of 25% ( Fig. 3b,c ), the maximum capacity is as high as ~1,675 mAh g −1 , corresponding to a lithiation potential of ~0.1 eV. Interestingly, presence of 25% DV defects was found to induce the formation of Li 3 C 8 at a relatively large potential of 0.84 eV, corresponding to a maximum capacity of 837 mAh g −1 . The favourable formation of Li 3 C 8 , as obtained through DFT calculations, coupled with the observation of an XRD peak corresponding to Li 3 C 8 in a fully lithiated graphene sample, provides compelling evidence for the formation of Li 3 C 8 clusters near DV defects in the graphene lattice. Such localized very-high lithium content intercalated states (formed in the vicinity of defects) could act as seed points for the subsequent plating of lithium metal as will be discussed later in this article. In the case of bulk metallic lithium (such as foils), non-uniformities in the structural morphology lead to a non-uniform current distribution [36] , [37] , [38] , [39] . This in turn leads to excessive localized charge densities and hence lithium metal tends to get non-uniformly plated, resulting in the formation of dendritic projections. A recent study [39] has shown that these structural non-uniformities originate not on the surface (as was originally thought) but in the sub-surface of the lithium electrode. Over extended cycling, these sub-surface dendrites burst out of the surface and protrude out into the electrolyte. The key point to be noted here is that conventional lithium metal foils lack pores or networks that can entrap dendrites that are formed in the sub-surface. Consequently, the dendritic projections are free to penetrate out of the surface and into the electrolyte, leading to potential shorting hazards. To illustrate this further we have included an SEM image ( Fig. 4a ) of the Li metal foil used in our testing, showing extensive dendritic formations on the surface. High-magnification SEM imaging of such dendritic structures has also been provided in the Supplementary Fig. 8 . By contrast the PGN anode ( Fig. 4b ) showed a conspicuous lack of such dendrites. 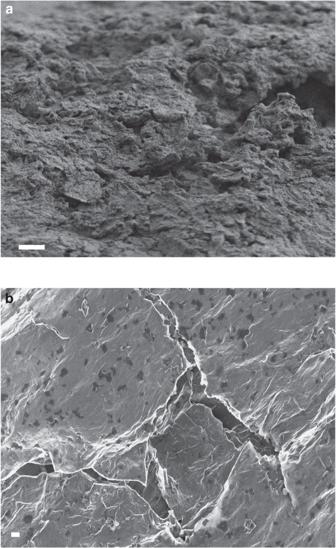Figure 4: Scanning electron microscopy characterization of the surface of the Li metal foils and the lithiated PGN. Top view SEM images of (a) lithium metallic foil showing significant roughness and morphological undulations along with sharp projections across the surface and (b) Li-PGN cathode showing the retention of the porous structure and no visible sharp edges or excessively rough features. Both the electrodes were run for 100 charge/discharge cycles at a rate of 5C. The cells were disassembled under a completely lithiated state. The scale bars in (a) and (b) are both 2 μm. Figure 4: Scanning electron microscopy characterization of the surface of the Li metal foils and the lithiated PGN. Top view SEM images of ( a ) lithium metallic foil showing significant roughness and morphological undulations along with sharp projections across the surface and ( b ) Li-PGN cathode showing the retention of the porous structure and no visible sharp edges or excessively rough features. Both the electrodes were run for 100 charge/discharge cycles at a rate of 5C. The cells were disassembled under a completely lithiated state. The scale bars in ( a ) and ( b ) are both 2 μm. Full size image For the PGN, it appears that the lithium plating is caused by formation of very-high lithium content intercalated states such as Li 3 C 8 at defect sites (divacancies) in the graphene lattice. It is well established that Li metal plating [2] , [3] , [4] , [36] , [37] , [38] , [39] is favored at sites that display large charge concentration (for example, concentration of lithium ions corresponding to Li 3 C 8 ). It is therefore reasonable to assume that the occurrence of Li 3 C 8 and Li metal are not unrelated. In our view the formation of Li 3 C 8 at defect sites in the graphene lattice seeds or initiates the Li metal plating. Hence, peaks for both Li 3 C 8 and Li metal can be observed in the XRD spectra for the lithiated PGN ( Fig. 2b ). So why does this Li plating for PGN not result in the formation of dendrites? Let us consider Li metal plating within the interior of the porous PGN electrode and its exterior surface. Within the interior of the electrode, Li metal plating occurs within pores that are few tens of nanometres in size (pore size distribution and SEM images of pore structure are provided in the Supplementary Figs 9,10 ). As a consequence, any dendritic structures associated with this plating will tend to remain confined within these pores due to its size constraints. However, it is noteworthy that even the exterior (outer) surface of the PGN electrode did not show any significant dendritic growth ( Fig. 4b ) even though there is no entrapment mechanism for Li that plates onto the exterior surface of the PGN. To understand this, we investigated the thickness of the plated Li on the exterior surface of the PGN. Our estimate for the maximum Li film thickness that plates onto the external PGN surface is ~5.8 nm (detailed calculations provided in the Supplementary Discussion ). The reason why this layer is so thin is that the exterior (outer) surface area of the PGN is very small when compared with the total surface area contained within the bulk of the porous PGN electrode. In other words, the porous PGN serves as a sponge that absorbs the majority of the Li metal into the interior of the electrode structure. The recent study by Harry et al. [39] shows that contrary to conventional wisdom dendrites are formed in the subsurface of Li foils, and not on the exterior surfaces as was previously thought. In fact, they found that the volume of the dendrite within the electrode is of the same order as the volume protruding into the electrolyte. For these reasons, the few-nanometre-thick Li film that plates onto the external surfaces of the PGN electrode will be unable to generate significant volumes of dendrites, which is consistent with our experimental observations. To further confirm the lack of dendrites on the exterior surfaces of the PGN, we performed SEM imaging for a lithiated PGN electrode that was tested for a prolonged time period (800 continuous charge/discharge cycles) at a C rate of ~1 C. The results ( Supplementary Fig. 11 ) also indicate the lack of dendrites on the outer (external) surface of the PGN electrode. In order to confirm the participation of the nano pores in entrapping lithium metal, scanning electron microscopy (SEM) images of PGN anodes were obtained under completely (a) lithiated and (b) delithiated conditions. SEM characterization techniques have often been employed to study plating and dendrite formation in lithium and are well accepted within the community [40] , [41] , [42] . 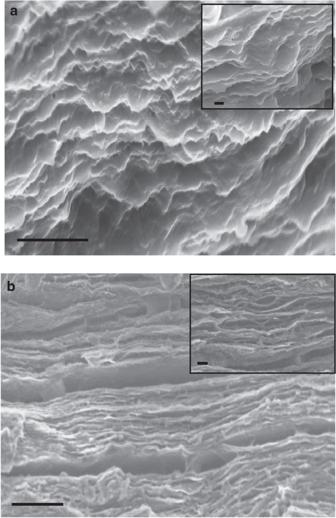Figure 5: Cross-sectional scanning electron microscopy characterization of the pore structure of the lithiated and delithiated PGN. (a) Cross-section SEM image of a completely lithiated PGN. The pores are visibly filled up and blocked by lithium metal. However, no dendritic projections could be observed. Inset shows a zoomed in image of the cross-section. (b) Cross-section SEM image of a completely delithiated PGN anode. The pores in this case have opened up once again, indicating that the plated lithium is indeed confined within these pores and that the lithiation–delithiation process is highly reversible. Inset shows a zoomed in image of the cross-section. The scale bar in (a) is 1 μm and in (b) it is 2 μm. The scale bars in the insets of (a) and (b) are both 200 nm. Figure 5a shows the cross section of PGN anode under a completely lithiated state (after the 1,000 th charge/discharge cycle). As is clearly visible, the pores are entirely filled up with lithium metal. Interestingly, no dendritic formations can be seen projecting out of the structure, even after 1,000 charge/discharge cycles, thereby allowing for operational safety. In contrast, the lithium metal foil used as the counter electrode showed significant dendritic structures, ranging in size from a few microns to tens of microns ( Supplementary Fig. 8 ). The reversibility of plated lithium and its ability to delithiate in the subsequent charge cycle can clearly be seen in Fig. 5b , whereby the cross-section of a PGN anode is shown under a completely delithiated state (after the 300 th charge/discharge cycle). The pores are seen to open up once again and are no longer filled with metallic lithium. From the cross-sectional SEM imaging in Fig. 5a,b we conclude that upon lithiation, the pores in the PGN tend to close (attributed to lithium plating that fills up the pore till it is finally constrained by the pore dimension) while upon delithiation, the lithium metal is released reversibly and the pores open up once again. These observations are further confirmed by the excellent cycle life of over 1,000 charge/discharge steps, with a coulombic efficiency of ~99% ( Fig. 1b ), thereby indicating a very impressive reversibility. These observations, along with the XPS profile of a completely delithiated sample showing the marked absence of lithium metal, address two critical issues that arise whenever there is an involvement of plating of lithium metal: (a) that the plated lithium metal is entrapped within the sub-surface of the PGN electrode and is therefore free from dendrite related problems and (b) the plating is highly reversible and does not tend to deteriorate the electrode–electrolyte interface or add to the loss of active lithium. Figure 5: Cross-sectional scanning electron microscopy characterization of the pore structure of the lithiated and delithiated PGN. ( a ) Cross-section SEM image of a completely lithiated PGN. The pores are visibly filled up and blocked by lithium metal. However, no dendritic projections could be observed. Inset shows a zoomed in image of the cross-section. ( b ) Cross-section SEM image of a completely delithiated PGN anode. The pores in this case have opened up once again, indicating that the plated lithium is indeed confined within these pores and that the lithiation–delithiation process is highly reversible. Inset shows a zoomed in image of the cross-section. The scale bar in ( a ) is 1 μm and in ( b ) it is 2 μm. The scale bars in the insets of ( a ) and ( b ) are both 200 nm. Full size image The steady rise in capacity over the first 300 cycles that we observe ( Fig. 1b ) can also be explained by the occurrence of lithium metal plating. During the first phase of cycling, the PGN anode undergoes volume expansion, as is observed in any graphitic anode. This in turn causes the pores within PGN to open up, thereby increasing its ability to store more metallic lithium and hence increasing the capacity with cycling. In addition, electrolytic access to all the DV defect sites might be limited during initial cycling owing to wettability characteristics of the PGN anode. As the cell is cycled, electrolyte wettability is enhanced and more defect sites are exposed for intercalation and subsequent plating reactions, further contributing to the rising capacity. This phenomenon continues until an equilibration stage is reached whereby the pores have completely opened up and the electrolyte completely wets the PGN anode. This is identified as the second phase of cycling (300 th cycle onwards) where a steady capacity of ~915 mAh g −1 is reached and is sustained throughout subsequent cycling ( Fig. 1b ). An important question that arises is—can we control the response of the PGN electrode by varying its state of defectiveness? To investigate this we performed a study in which we varied the thermal reduction time for a fixed thickness of the PGN electrode. In this test, free-standing GO papers (~20 μm thick) were exposed to a thermal shock at ~700 °C for ~45 s, ~60 s and ~75 s respectively. Raman spectra of the PGN electrodes indicated a significant increase in defect density (quantified by the I D / I G ratio) with increasing reduction time (see Supplementary Fig. 12a ). This shows that it is possible to control the thermal reduction parameters to tune the state of defectiveness of the PGN electrode. The PGN electrodes with varying levels of defectiveness were tested as anode materials in coin cells. The results ( Supplementary Fig. 12b ) show a strong correlation between the state of defectiveness and the specific capacities of the PGN. The higher the state of defectiveness, the higher the measured charge storage capacities of the electrodes. This is consistent with our DFT model, since PGN electrodes that are more defective will have greater density of DV sites that act as seed points to initiate Li metal plating. Therefore, more defective samples show significantly greater Li capacities as opposed to the less-defective samples. In order to control the PGN electrode’s performance it is important to recognize that the optimal thermal reduction parameters also depend on the thickness of the GO paper that is being reduced. In Fig. 1 , the optimal thermal reduction time was ~45 s, because the thickness of the GO paper was only ~10 μm as opposed to ~20 μm for the samples tested in Supplementary Fig. S12a,b . Galvanostatic discharge–charge curves of PGN with different amount of defects is provided in the Supplementary Fig. 12c . In this figure, we have also compared the voltage profile of PGN anodes with traditional graphitic anodes [43] . Graphitic anodes generally show a characteristic voltage plateau ( Supplementary Fig. S12c ) below 250 mV during both charge and discharge cycles [43] , [44] , [45] . This phenomenon in graphite is attributed to the standard stage I formation of LiC 6 intercalates during lithiation and the extraction of Li from LiC 6 intercalates during delithiation, each step corresponding to charge/discharge capacities [45] of ~372 mAh g −1 . However, in comparison, the voltage profiles of PGN anodes are significantly different from that of graphitic carbon. Unlike graphitic carbon, there is a marked absence of a single voltage plateau below 250 mV. Instead, the presence of a gradual slope below 1 V during discharge and above 1 V during charge indicates that the primary reaction mechanism for the PGN is different from the conventional LiC 6 intercalation observed in graphite. Given the evidence of lithium metal peaks in XRD as well as XPS analysis carried out on fully Lithiated PGN anodes, we conclude that the primary reaction mechanism is lithium metal plating, whereby Li 3 C 8 acts as seed points to increase the localized charge density and initiate the plating mechanism. The mechanism of defect-induced storage of metallic lithium within a porous structural network was then extended to synthesize a high-performance cathode material. Lithium metal offers the highest theoretical capacity (3,842 mAh g −1 ) in lithium ion batteries [43] and a cathode material comprising lithium metal would thus be most suitable for next-generation high-energy-density batteries. In order to develop a facile method for cathode synthesis, it was decided to cycle a regular PGN anodic half cell to initiate the natural intercalation and plating steps. This would be followed by disassembling the anodic half cell (in a completely lithiated state) and reassembling it into a cathodic half cell ( Fig. 6a ). However, a critical road-block to this approach was the time required for fabrication of such a cathode. At a rate of 1C, thermally reduced PGN anodes took ~300 cycles to reach a stable capacity in excess of 900 mAh g −1 and would thus not be a suitable method for cathode fabrication. Following the theoretical DFT calculations and its analysis however, it was evident that the presence of an opened-up graphene network with a greater density of defects would allow for (a) better electrolyte wettability and (b) more defect sites for seed formation. This in turn would ensure that the high capacities were reached faster and the anodic half cell could be disassembled earlier. Therefore, an alternate approach of flash reduction was carried out to prepare PGN anodes that would then be cycled at 1 C for a fixed time before being disassembled and reassembled as a cathodic half cell. 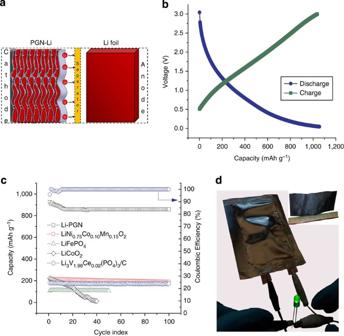Figure 6: Lithiated-PGN cathodes for high-capacity lithium-ion batteries. (a) Schematic representation of the cathodic half cell constructed with the PGN electrode containing lithium metal within its pores. (b) Voltage profile of the cathodic half cell indicating an efficient lithiation–delithiation process. (c) Capacity and coulombic efficiency versus cycle index of lithium/PGN cathodes at a charge/discharge rate of ~1C (current density of ~0.3 Ag−1). For comparison, the capacity versus cycle index achievable from various cathode materials (namely LiCoO2, LiFePO4, LiNi0.75Co0.10Mn0.15O2and Li3V1.98Ce0.02(PO4)3/C) measured at comparable current densities has been included in the figure (taken from refs47,48,49,50). (d) Macroscopic pouch cell (full-cell configuration) of PGN anode and Li-PGN cathode shown here powering an LED device. Since exclusively carbon based materials are used for electrode construction, the only active source of lithium in the full-cell is the lithium metal that is entrapped within the pores of the PGN cathode. The pouch cell had a capacity rating of ~20 mAh. Inset shows a photograph of a large-scale GO paper measuring ~30 cm2in area and ~100 μm in thickness that was used to construct the PGN and Li-PGN electrodes for the pouch cell. Figure 6: Lithiated-PGN cathodes for high-capacity lithium-ion batteries. ( a ) Schematic representation of the cathodic half cell constructed with the PGN electrode containing lithium metal within its pores. ( b ) Voltage profile of the cathodic half cell indicating an efficient lithiation–delithiation process. ( c ) Capacity and coulombic efficiency versus cycle index of lithium/PGN cathodes at a charge/discharge rate of ~1C (current density of ~0.3 Ag −1 ). For comparison, the capacity versus cycle index achievable from various cathode materials (namely LiCoO 2 , LiFePO 4 , LiNi 0.75 Co 0.10 Mn 0.15 O 2 and Li 3 V 1.98 Ce 0.02 (PO 4 ) 3 /C) measured at comparable current densities has been included in the figure (taken from refs 47 , 48 , 49 , 50 ). ( d ) Macroscopic pouch cell (full-cell configuration) of PGN anode and Li-PGN cathode shown here powering an LED device. Since exclusively carbon based materials are used for electrode construction, the only active source of lithium in the full-cell is the lithium metal that is entrapped within the pores of the PGN cathode. The pouch cell had a capacity rating of ~20 mAh. Inset shows a photograph of a large-scale GO paper measuring ~30 cm 2 in area and ~100 μm in thickness that was used to construct the PGN and Li-PGN electrodes for the pouch cell. Full size image Photo-thermal (or flash) reduction has been demonstrated as a viable method for reduction of GO by our group [46] . While previously the flash reduction was performed by a relatively low-energy digital camera, in this case the flash reduction was carried out using a controllable studio Xenon flash (Einstein E640) at a very high energy of ~320 Ws in order to induce wider pore formation and greater density of defect sites (cross-section SEM images are included in the Supplementary Fig. 13 ). Interestingly, the flash-reduced PGN anode stabilized to a capacity >1,000 mAh g −1 at a rate of 1 C in <10 cycles of operation, which ensures that the PGN gets fully lithiated in less than a day. At this stage, the anode was disassembled in a completely lithiated state inside a glove box and its mass was recorded in a microgram weighing balance. The lithiated PGN was then reassembled into a cathodic half cell. The mass loading of the cathode was ~1 mg cm −2 , which is comparable to the industrial standard for commercial Li-ion batteries. The lithiated PGN cathode was cycled between 0.03 V and 3.2 V at a constant current density of ~300 mA g −1 and a specific capacity in excess of 850 mAh g −1 (based on the total mass of lithium+PGN) was observed, stable over 100 cycles, corresponding to an energy density of ~637 Wh kg −1 and a power density of ~200 W kg −1 . The voltage profile indicated smooth lithiation and delithiation profiles, as shown in Fig. 6b . By contrast, the practically realizable capacities and energy densities for LiMnO 2 , LiFePO 4 and LiCoO 2 cathodes lie [12] , [13] , [14] in the 110–170 mAh g −1 and 470–545 Wh kg −1 range, respectively. A comparison of the specific capacities versus cycle index obtained from the lithiated PGN cathode and conventional cathode materials [47] , [48] , [49] , [50] has been provided in Fig. 6c . A comparison of the working voltage, achievable capacities and practical energy densities of conventional anode and cathode materials as well as PGN anodes and lithiated PGN cathodes has been provided in Table 1 . To demonstrate the versatility and scalability of the PGNs, we assembled a full-cell (in a macroscopic pouch cell configuration- Fig. 6d ) with PGN anodes and lithiated PGN (Li-PGN) cathodes, stacked to provide an ampere-hour rating of ~20 mAh. The inset in Fig. 6d shows a photograph of a free-standing GO paper with an area of ~30 cm 2 and a thickness of ~100 μm. This GO paper was cut into electrodes (~5 cm 2 in area) and reduced using a Xenon flash (Einstein E640, energy—320 Ws). These individual ~5-cm 2 electrodes were then used to construct the pouch cell stack and demonstrated a mass loading of ~2.5 mg cm −2 , well within the industrial standards of 1–5 mg cm −2 . The pouch cell was successfully used to power an LED device, as shown in the photograph. This particular pouch cell comprised a stack of three full cells; however, the ampere-hour rating can be increased by adding more cells to the stack or by simply increasing the area of each cell. It should be noted that the full-cell (with PGN electrodes) demonstrated in Fig. 6d operates on the well-established principle of transfer of Li ions back and forth between the cathode and anode material. In this regard this concept is no different from a conventional Li-ion battery. What is different is that the electrode material that stores the Li is all-carbon for both the anode as well as the cathode. Therefore the electrodes in our Li-ion full-cell configuration are exclusively made from carbon (PGN) materials into which Li ions are reversibly plated and stored. To conclude, we have demonstrated a new mechanism of defect-induced plating of lithium metal in PGNs. The graphene network not only acts as a caged entrapment for lithium metal (that prevents dendritic growth) but also provides a conductive network for efficient electron transfer (no current collectors are used), thereby offering significant improvements over other less-conductive cathodes that often require additional doping [47] . The successful demonstration of a pouch cell (in a full-cell configuration) with PGN anodes and Li-PGN cathodes indicates the feasibility of an all-carbon lithium battery, which could greatly simplify the battery chemistry. Finally, the demonstration of a macroscopic pouch cell indicates the feasibility of scale-up, which is a concern for nanostructured electrodes that often lack sufficient active mass [18] to build a viable battery. Preparation of GO paper GO dispersed in de-ionized water (ACS materials—10 mg ml −1 ) was diluted to concentrations of ~1 mg ml −1 and sonicated in a Bransonic 1510MT ultrasonic cleaner for ~1 h to ensure homogenous dispersion and centrifuged in a Sorvall Legend XTR Centrifuge (Thermo Fisher Scientific) at ~6,000 r.p.m. for ~30 min to ensure removal of heavier aggregates. GO papers were prepared by vacuum filtration. Briefly, ~50 ml of the supernatant GO solution were passed through ~0.2-μm pore size Whatman Anodisc filters (47 mm diameter) to prepare papers of ~10–20 μm thicknesses, which were then carefully peeled off the filter and stored in a desiccator till further use. For thicker GO papers (80–100 μm range), we used electro-deposition as opposed to vacuum filtration to reduce the deposition time. In this method, the GO colloidal solution in water was placed between two electrodes and a potentiostatic field (constant DC voltage of ~10 V) was applied. Thick GO films could be rapidly deposited on the surface of the working electrode (Al foil) by this method and then peeled off the Al surface. Preparation of PGN electrodes In order to prepare PGN anodes, the GO paper was placed in a ~1-inch diameter quartz tube with an argon flow of ~500 sccm at atmospheric pressure. The sample was then rapidly introduced into a Thermolyne 79300 tube furnace kept at ~700 °C, and held for ~45 s. The rapid heating induces deoxygenation of the GO sheets to produce a binder-free structurally stable PGN paper. The optimal reduction time is found to be sensitive to the thickness of the precursor GO paper. For ~10-μm thick GO paper the optimal reduction time is ~45 s, but increases to ~75 s for ~20-μm thick GO paper. Battery testing PGN anodes and lithium/PGN cathodes were tested as anodic and cathodic half cells respectively in 2032 coin cells. The cells were assembled inside a glove box (MBraun Labstar) with oxygen and moisture content <1 p.p.m. Lithium foil was used as the counter electrode and a Celgard 2340 polypropylene membrane was used as the separator. The electrolyte was 1 M LiPF 6 in 1:1 mixture of ethylene carbonate (EC) and diethyl carbonate (DEC). The electrolyte and lithium metal foil were purchased from Novolyte and FMC Lithium, respectively. An Arbin BT2000 Battery Tester was used to run the charge/discharge cycles. Characterization of PGN electrodes Disassembly of the coin cells for characterization and re-assembly as cathodes was carried out inside the glove box. For characterization, the PGN anode was soaked in dimethyl carbonate overnight to remove excess electrolyte. Owing to the relatively low penetration depth of XPS, the top surface of the PGN was partially removed by using the scotch tape method. This resulted in exposing the interior of the electrode for characterization purposes. The sample preparation was carried out after drying the electrodes overnight. Following the sample preparation and overnight drying step, the materials were transported in an argon-filled gas-tight container for XPS, XRD and SEM characterizations. The container was briefly opened to transfer the material into the equipment chamber (in the case of XPS and SEM) before pumping it down to vacuum once again. Cathode half cells were assembled without removing the solid electrolyte interface layer and the entire process was carried out entirely inside the glove box. Pouch cell assembly Macroscopic pouch cell configurations were assembled inside the glove box. For synthesis of Li-PGN, the pouch cell comprised stacked PGN anodes against lithium foil as the counter electrode, separated by a Celgard 2340 polypropylene membrane. The electrolyte was 1 M LiPF 6 in EC:DEC. The individual cells were insulated from the rest of the stack to avoid any potential shorting through an insulating membrane separator. Sealing was achieved by means of a heat sealer. The pouch cell was taken out of the glove box for cycling following the sealing step and cycled to achieve lithiation. Once lithiation of the PGN anode was achieved, the pouch cell was reopened inside the glove box and the lithiated PGN electrodes were recovered and re-assembled as cathodes into a full-cell configuration against pristine PGN anodes, following the same steps as mentioned above. Theoretical calculations Theoretical calculations were performed using the Vienna Ab Initio Simulation Package (VASP) with the projector-augmented wave method and the Perdew–Burke–Ernzerhof form of the generalized gradient approximation for exchange and correlation. For convergence studies, we determined a kinetic energy cutoff of 600 eV and a Fermi smearing width of 0.05 eV. The Brillouin zones of 4 × 4 and 5 × 5 supercell are sampled with the Γ-centred k-point grid of 9 × 9 × 1 and 7 × 7 × 1, respectively. In order to avoid the spurious coupling effect between graphene layers along the z axis, the vacuum separation in the model structure is set to 18 Å. All atoms and cell-vectors are relaxed with a force tolerance of 0.02 eV. The lithiation potential V is defined as where the change in Gibb’s free energy is Since the term PΔV f is of the order of 10 −5 eV, whereas the term TΔS f is of the order of the thermal energy (26 meV at room temperature), the entropy and the pressure terms can be neglected and the free energy will be approximately equal to the formation energy ΔE f obtained from DFT calculations. The formation energy is defined as where n is the number of lithium atoms inserted in the computational cell, is the total energy of the lithiated graphene ( Li n G ) structure, E Li is the total energy of a single lithium atom in elemental body-centred cubic lithium, and E G is the total energy of a particular graphene structure. From DFT calculation, we have obtained E Li to be −1.8978, eV. If the energies are expressed in electron volts, the potential of the Li n G structures versus Li/Li + as a function of lithium content can be obtained as The composition range over which lithium can be reversibly intercalated determines the battery capacity. How to cite this article: Mukherjee, R. et al. Defect-induced plating of lithium metal within porous graphene networks. Nat. Commun. 5:3710 doi: 10.1038/ncomms4710 (2014).